Laser-induced porous graphene films from commercial polymers The cost effective synthesis and patterning of carbon nanomaterials is a challenge in electronic and energy storage devices. Here we report a one-step, scalable approach for producing and patterning porous graphene films with three-dimensional networks from commercial polymer films using a CO 2 infrared laser. The sp 3 -carbon atoms are photothermally converted to sp 2 -carbon atoms by pulsed laser irradiation. The resulting laser-induced graphene (LIG) exhibits high electrical conductivity. The LIG can be readily patterned to interdigitated electrodes for in-plane microsupercapacitors with specific capacitances of >4 mF cm −2 and power densities of ~9 mW cm −2 . Theoretical calculations partially suggest that enhanced capacitance may result from LIG’s unusual ultra-polycrystalline lattice of pentagon-heptagon structures. Combined with the advantage of one-step processing of LIG in air from commercial polymer sheets, which would allow the employment of a roll-to-roll manufacturing process, this technique provides a rapid route to polymer-written electronic and energy storage devices. Over the past decade, graphene-based nanomaterials have been widely studied owing to their unique physical and chemical properties [1] . Through synthesis and engineering design, graphene can have porous and three-dimensional (3D) structures, leading to a wide range of applications from composite fillers to energy storage devices [2] , [3] . Despite the tremendous advances, current synthesis methods of porous graphene require either high temperature processing [2] , [3] , [4] , or multi-stepped chemical synthesis routes [5] , [6] , [7] , lessening their wide-spread commercial potential. Therefore, straightforward synthesis, and especially patterning, of graphene-based nanomaterials in a scalable approach is still a technologically important goal in achieving commercialized microscale energy storage devices, and in particular for emerging wearable electronics [8] . Glassy carbon has been produced from insulating polyimide (PI) via pulsed ultraviolet laser treatment [9] . However, to our knowledge, the detailed structural study of the obtained materials, especially at the near-atomic level; the correlation of the material structures to their electrochemical performance, and the formation of graphene by this route have not been disclosed. Moreover, the technique of laser scribing on insulating polymers for the fabrication of microsupercapacitors (MSCs) has not hitherto been demonstrated. In this work, we demonstrate the production of 3D porous graphene films from polymers by laser induction. The materials are well characterized and demonstrate a new application in energy storage. Moreover, theoretical calculations provide support for the proposed mechanism of enhanced charge storage in correlation with analytical results from high-resolution imaging. Laser scribing As depicted in Fig. 1a , irradiation of a commercial PI film by a CO 2 infrared laser under ambient conditions converts the film into porous graphene which we term laser-induced graphene (LIG) ( Supplementary Fig. 1a ). With computer-controlled laser scribing, LIG can be readily written into various geometries, as shown in the scanning electron microscopy (SEM) image in Fig. 1b . The photographs in Supplementary Figs 1b,c show two distinguished areas: black LIG after PI was exposed to the laser, and light orange PI that was unexposed. We [10] and other groups [11] , [12] , [13] , [14] , [15] , [16] have recently demonstrated fabrication of MSCs using conventional lithography techniques that require masks and restricted-operational conditions. While there have been some recent developments in laser scribing of hydrated graphene oxide (GO) films [17] , [18] , here we show a one-step laser scribing on commercial polymer films in air to form 3D-graphene layers. The approach is inherently scalable and cost-effective in fabricating large-area devices ( Supplementary Movie 1 ), and might be transferred to a roll-to-roll process. 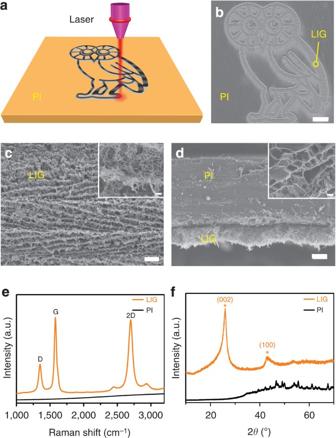Figure 1: LIG formed from commercial PI films using a CO2laser at a power of 3.6 W to write patterns. (a), Schematic of the synthesis process of LIG from PI. (b), SEM image of LIG patterned into an owl shape; scale bar, 1 mm. The bright contrast corresponds to LIG surrounded by the darker-colored insulating PI substrates. (c), SEM image of the LIG film circled in (b); scale bar, 10 μm. Inset is the corresponding higher magnification SEM image; scale bar, 1 μm. (d), Cross-sectional SEM image of the LIG film on the PI substrate; scale bar, 20 μm. Inset is the SEM image showing the porous morphology of LIG; scale bar, 1 μm. (e), Representative Raman spectrum of a LIG film and the starting PI film. (f), XRD of powdered LIG scraped from the PI film. Figure 1: LIG formed from commercial PI films using a CO 2 laser at a power of 3.6 W to write patterns. ( a ), Schematic of the synthesis process of LIG from PI. ( b ), SEM image of LIG patterned into an owl shape; scale bar, 1 mm. The bright contrast corresponds to LIG surrounded by the darker-colored insulating PI substrates. ( c ), SEM image of the LIG film circled in ( b ); scale bar, 10 μm. Inset is the corresponding higher magnification SEM image; scale bar, 1 μm. ( d ), Cross-sectional SEM image of the LIG film on the PI substrate; scale bar, 20 μm. Inset is the SEM image showing the porous morphology of LIG; scale bar, 1 μm. ( e ), Representative Raman spectrum of a LIG film and the starting PI film. ( f ), XRD of powdered LIG scraped from the PI film. Full size image Analytical characterization LIG films obtained with a laser power of 3.6 W, denoted as LIG-3.6 W, were further characterized with SEM, Raman spectroscopy, X-ray diffraction (XRD), X-ray photoelectron spectroscopy (XPS) and Fourier-transform infrared spectroscopy. Figure 1c shows that LIG films exhibit the appearance of a foam with porous structures resulting from the rapid liberation of gaseous products [19] . Cross-sectional SEM images of LIG reveal ordered-porous morphology ( Fig. 1d ). These porous structures render enhanced-accessible surface areas and facilitate electrolyte penetration into the active materials. The Raman spectrum of LIG ( Fig. 1e ) shows three prominent peaks: the D peak at ~1,350 cm −1 induced by defects or bent sp 2 -carbon bonds, the first-order allowed G peak at ~1,580 cm −1 and the 2D peak at ~2,700 cm −1 originating from second order zone-boundary phonons [20] . If PI is carbonized at temperatures ranging from 800 to 1,500 °C, the resulting Raman spectrum is similar to that of glassy carbon ( Supplementary Fig. 2 ). But the spectrum for LIG ( Fig. 1e ) is clearly different from that of glassy carbon [21] . The 2D peak of LIG can be fitted with only one Lorentzian peak centred at 2,700 cm −1 , the same as in single-layer graphene [20] , but with a larger full width at half maximum of ~60 cm −1 . This 2D band profile is typical of that found in 2D graphite consisting of randomly stacked graphene layers along the c axis [22] , [23] . Finally, D/G intensity ratio indicates a high degree of graphene formation in the LIG films [20] . The XRD pattern ( Fig. 1f ) shows an intense peak centred at 2 θ =25.9°, giving an interlayer spacing ( I c ) of ~3.4 Å between (002) planes in the LIG, and it indicates the high degree of graphitization. The asymmetry of the (002) peak, with tailing at smaller 2 θ angles, also points to an increased I c . The expanded I c can be attributed to regions where defects are distributed on hexagonal graphene layers. The peak at 2 θ =42.9° is indexed to (100) reflections which are associated with an in-plane structure. Using equations (2) and (3) (Methods), the crystalline size along the c axis (L c ) and a axis (L a ) are calculated to be ~17 nm and ~32 nm, respectively. The XPS spectrum of LIG-3.6 W shows a dominant C—C peak with greatly suppressed C—N, C—O and C=O peaks ( Supplementary Fig. 3 ). It suggests that LIG films are dominated by sp 2 -carbons, agreeing well with the Raman and XRD results. This is further confirmed by comparison of the distinctive Fourier-transform infrared spectra of PI and LIG-3.6 W ( Supplementary Fig. 4 ). The micro and nano structure of LIG flakes was investigated by transmission electron microscopy (TEM). Supplementary Fig. 5a shows thin LIG flakes with few-layer features, as further indicated, from the edges of the flake in Fig. 2a . Moreover, ripple-like wrinkled structures can be observed from the surface of the flakes; these structures in graphene have been shown to improve the electrochemical performance of devices [24] . Thicker flakes exhibit mesoporous structures ( Supplementary Fig. 5b ). High-resolution TEM image in Fig. 2b reveals that the nano-shaped ripples are exposed edges of graphene layers. The formation of these ripples could be attributed to thermal expansion caused by laser irradiation. The average lattice space of ~3.4 Å shown in Fig. 2b corresponds to the distance between two neighbouring (002) planes in graphitic materials, and it agrees well with the XRD results. The aberration-corrected scanning TEM (Cs-STEM) image ( Fig. 2c ) shows the unusual ultra-polycrystalline feature of LIG flakes with disordered-grain boundaries. This observation is further depicted in Fig. 2d , expanding a hexagon lattice with a heptagon with two pentagons. These abundant pentagon-heptagon pairs can account for the curvature of the graphene layers leading to the porous structure [25] ( Supplementary Figs 5c,d and 6 ). Importantly, these defects could offer avenues towards functionalization of LIG for catalysis applications [26] . In addition, our theoretical calculations suggest that these defects could enhance electrochemical capacity, and this will be discussed in detail below. LIG has a surface area of ~340 m 2 ·g −1 by BET, with pore sizes <9 nm ( Supplementary Fig. 7 ). Thermogravimetric-analysis measurement under argon ( Supplementary Fig. 8 ) shows that the decomposition temperature of PI is ~550 °C and LIG is >900 °C, whereas that of the often used graphene precursor, GO, is ~190 °C. 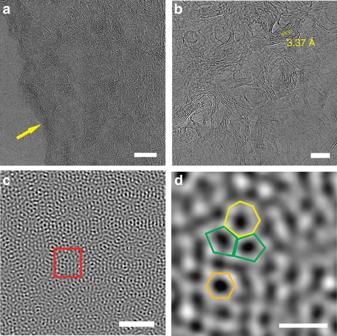Figure 2: TEM images of LIG obtained with a laser power of 3.6 W. (a), High-resolution TEM (HRTEM) image taken at the edge of a LIG flake showing few-layer features and highly-wrinkled structures; scale bar, 10 nm. (b), HRTEM image of LIG; scale bar, 5 nm. Average lattice space of ~3.4 Å corresponds to the (002) planes of graphitic materials. (c), Cs-STEM image taken at the edge of a LIG flake; scale bar, 2 nm. It shows an ultra-polycrystalline nature with grain boundaries. (d), TEM image of selected area indicated as a rectangle in (c). It shows a heptagon with two pentagons, as well as a hexagon; scale bar, 5 Å. Figure 2: TEM images of LIG obtained with a laser power of 3.6 W. ( a ), High-resolution TEM (HRTEM) image taken at the edge of a LIG flake showing few-layer features and highly-wrinkled structures; scale bar, 10 nm. ( b ), HRTEM image of LIG; scale bar, 5 nm. Average lattice space of ~3.4 Å corresponds to the (002) planes of graphitic materials. ( c ), Cs-STEM image taken at the edge of a LIG flake; scale bar, 2 nm. It shows an ultra-polycrystalline nature with grain boundaries. ( d ), TEM image of selected area indicated as a rectangle in ( c ). It shows a heptagon with two pentagons, as well as a hexagon; scale bar, 5 Å. Full size image Effect of laser power To investigate the effect of laser power, LIG was prepared using powers ranging from 2.4 W to 5.4 W in 0.6 W increments at a scan rate of 3.5 inches s −1 . In Fig. 3a (plotted from Supplementary Table 1 ), beginning at 2.4 W, the atomic percentage of carbon sharply increases from the original 71% in PI to 97% in LIG whereas the atomic percentages of both nitrogen and oxygen decrease precipitously to <3%. This threshold-power effect has been well-studied in ultraviolet ablation of polymers [27] . The threshold power shows a linear dependence on the scan rate ( Supplementary Fig. 9 ). If the scan rate increases, higher threshold power needs to be applied in order to initiate the graphitization. Meanwhile, the sheet resistance (R s ) of LIG-2.4 W is reduced to <35 Ω per square ( Fig. 3b ). Below the threshold of 2.4 W, PI is an insulator with R s >90 MΩ per square (instrument limit). As the laser power increases to 5.4 W, R s is gradually reduced to a minimum value of <15 Ω per square; the translated conductivity is ~25 S cm −1 , higher than in laser-reduced GO [28] . 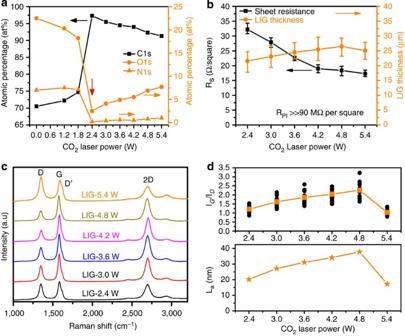Figure 3: Characterizations of LIG prepared with different laser powers. (a), Atomic percentages of carbon, oxygen and nitrogen as a function of laser power. These values are obtained from high-resolution XPS. The threshold power is 2.4 W, at which conversion from PI to LIG occurs. (b), Correlations of the sheet resistance and LIG film thicknesses with laser powers. (c), Raman spectra of LIG films obtained with different laser powers. (d), Statistical analysis of ratios of G and D peak intensities (upper panel), and average domain size alongaaxis (La) as a function of laser power (xaxis) calculated using equation (4). Figure 3b shows two distinct slopes of Rs versus laser power. The slope when the laser power was <4.2 W is larger than the one when it was >4.2 W. This suggests that when the laser power is <4.2 W, the thermal power dominates the quality of the films. Therefore, increased laser power leads to higher degree of graphitization. As the thermal power rises above 4.2 W, oxidation starts to play an increasingly deleterious role in the quality of the films. Therefore the slope lessens. Figure 3: Characterizations of LIG prepared with different laser powers. ( a ), Atomic percentages of carbon, oxygen and nitrogen as a function of laser power. These values are obtained from high-resolution XPS. The threshold power is 2.4 W, at which conversion from PI to LIG occurs. ( b ), Correlations of the sheet resistance and LIG film thicknesses with laser powers. ( c ), Raman spectra of LIG films obtained with different laser powers. ( d ), Statistical analysis of ratios of G and D peak intensities (upper panel), and average domain size along a axis (L a ) as a function of laser power ( x axis) calculated using equation (4). Full size image As expected, higher laser power tends to increase porosity, as shown in the SEM images taken on the backsides of the LIG films ( Supplementary Fig. 10 ) that had been peeled off the PI substrates. Raman spectroscopy is a powerful tool to obtain crystalline size (L a ) along the a axis of graphitic materials by analyzing ratios of the integrated intensities of G and D peaks (I G /I D ) [29] . Figure 3c shows representative Raman spectra of LIG films attained with laser powers from 2.4 W to 5.4 W. The statistical analysis of I G /I D versus laser powers is plotted in the upper panel of Fig. 3d . The L a values calculated from the average I G /I D ratio using equation (4) (Methods) is shown in the lower panel of Fig. 3d , showing increased L a up to ~40 nm as the laser power rises to 4.8 W. This increase can be attributed to increased surface temperatures [27] . Further increase in power degrades the quality of the LIG with L a of ~17 nm in LIG-5.4 W, which is attributable to the partial oxidation of LIG in air. This can be further verified from profound defect-correlated D peaks centred at ~1,620 cm −1 in LIG-5.4 W ( Fig. 3c ). Laser ablation of polymers has been studied since the early 1980s ref. 30 . Because of its complex nature, the detailed mechanism is still debated as being a photothermal or photochemical process, or both [31] . Since photochemical processes tends to occur in lasers with short wavelengths and ultra-short pulse widths, our infrared LIG formation is more likely to be caused by photothermal effects owing to the long wavelength (~10.6 μm) and relatively long pulses (~14 μs) of the CO 2 laser. The energy from laser irradiation results in lattice vibrations which could lead to extremely high localized temperatures (>2,500 °C) that can be qualitatively detected by laser-induced fluorescence ( Supplementary Movie 1 ) [19] . This high temperature could easily break the C—O, C=O and N—C bonds, as confirmed by the dramatically decreased oxygen and nitrogen contents in LIG ( Fig. 3a ). These atoms would be recombined and released as gases. Aromatic compounds are then rearranged to form graphitic structures, during which oxidation of these graphitic structures can be minimized by an overlayer of the evolved gases. We have found that the mechanism of laser graphitization in polymers is strongly correlated to the structural features present in the repeat units, such as aromatic and imide repeat units. We tried to generalize this laser-induced graphitization process by testing 15 different polymers. Out of them, only two polymers, PI and poly(etherimide), both of which contain aromatic and imide repeat units, can form LIG ( Supplementary Table 2 and Supplementary Fig. 11 ). Four other step-growth polymers and all nine of the chain-growth polymers tested did not afford LIG. The reason for other step-growth polymers being inactive is not conclusively known. The chain-growth polymers likely undergo rapid depolymerization at the laser-induced temperatures. Inspired by the advantages suggested from the experimental results, we fabricated in-plane interdigitated LIG microsupercapacitors (LIG-MSCs) in which LIG serves as both the active electrodes and the current collectors. Well-defined LIG-MSC electrodes are directly written on PI sheets with a neighbouring distance of ~300 μm ( Fig. 4a,b ). This distance can be further decreased by using a smaller laser aperture. After writing, silver paint was applied on common positive and negative electrodes, and then Kapton tape was employed to define the active electrodes. 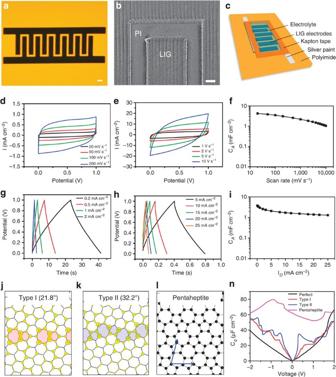Figure 4: Electrochemical performances of LIG-MSC devices from LIG-4.8 W in 1 M H2SO4with their GB-induced properties. (a), A digital photograph of LIG-MSCs with 12 interdigital electrodes; scale bar, 1 mm. (b), SEM image of LIG electrodes; scale bar, 200 μm.c, Schematic diagram of LIG-MSCs device architecture. (dande), CV curves of LIG-MSCs at scan rates from 20 to 10,000 mV s−1. (f), Specific areal capacitance (CA) calculated from CV curves as a function of scan rates. (gandh), CC curves of LIG-MSCs at discharge current densities (ID) varied from 0.2 to 25 mA cm−2. (I), CAcalculated from CC curves versus ID. (jandk), Charge density distribution of the states within a voltage window (−0.1, 0.1) V for type I and II polycrystalline sheets. The defects at the grain boundaries are shadowed, and numbers show the misorientation angle between the grains. (l), A carbon layer fully composed of pentagons and heptagons (pentaheptite). (n), Calculated quantum capacitance (defined in the text) of perfect and polycrystalline/disordered graphene layers. Figure 4c depicts the device architecture of the fabricated LIG-MSCs, and the fabrication protocol is described in the Methods. Cyclic voltammetry (CV) and galvanostatic charge-discharge (CC) measurements were then performed to investigate the electrochemical performance of the fabricated LIG-MSCs. All CV curves of LIG-MSCs made with LIG electrodes at various laser powers are pseudo-rectangular in shape, which indicates good double-layer capacitive behaviours ( Supplementary Fig. 12a ). LIG-MSCs constructed with LIG-4.8 W electrodes generally exhibit the highest specific areal capacitance ( C A ; Supplementary Fig. 12b ). The C A of LIG-MSCs made from poly(etherimide) is ~10% of those from PI ( Supplementary Fig. 12c-d ), possibly associated with the lower nitrogen content. Therefore, all other electrochemical measurements were carried out on LIG-MSCs made from PI with a laser power of 4.8 W. Figures 4d–e are the CV curves at scan rates ranging from 20 to 10,000 mV s −1 . Although, there exist certain level of oxygen or nitrogen contents in LIG, the devices do not exhibit pseudo-capacitive behaviour as suggested from CV curve at small rate of 20 mV s −1 which shows no anodic and cathodic peaks. Even at a high rate of 10,000 mV s −1 , the CV curve maintains its pseudo-rectangular shape, and this is suggestive of high-power performance. The C A as a function of scan rate is shown in Fig. 4f . At a scan rate of 20 mV s −1 , the C A is >4 mF cm −2 which is comparable with or higher than the values obtained in recently reported GO-derived supercapacitors [6] , [13] , [17] , [18] , [32] ; the specific capacitance of the material by weight is ~120 F g −1 . At 10,000 mV s −1 , the C A is still higher than 1 mF cm −2 . This excellent capacitive behaviour is further confirmed by the nearly triangular CC curves at varying current densities from 0.2 to 25 mA·cm −2 ( Fig. 4g–h ). From the C A versus discharge current densities (I D ) plotted in Fig. 4i , the LIG-MSCs can deliver C A of ~3.9 mF cm −2 at I D of 0.2 mA cm −2 and still maintain 1.3 mF cm −2 even when the devices are operated at I D of 25 mA cm −2 . This value is comparable or higher than those reported for some carbon-based MSCs at the same current densities [12] , [13] , [17] , [18] . The impedance measurement shows a low-equivalent series resistance of 7 Ω ( Supplementary Fig. 13 ). Figure 4: Electrochemical performances of LIG-MSC devices from LIG-4.8 W in 1 M H 2 SO 4 with their GB-induced properties. ( a ), A digital photograph of LIG-MSCs with 12 interdigital electrodes; scale bar, 1 mm. ( b ), SEM image of LIG electrodes; scale bar, 200 μm. c , Schematic diagram of LIG-MSCs device architecture. ( d and e ), CV curves of LIG-MSCs at scan rates from 20 to 10,000 mV s −1 . ( f ), Specific areal capacitance (C A ) calculated from CV curves as a function of scan rates. ( g and h ), CC curves of LIG-MSCs at discharge current densities (I D ) varied from 0.2 to 25 mA cm −2 . ( I ), C A calculated from CC curves versus I D . ( j and k ), Charge density distribution of the states within a voltage window (−0.1, 0.1) V for type I and II polycrystalline sheets. The defects at the grain boundaries are shadowed, and numbers show the misorientation angle between the grains. ( l ), A carbon layer fully composed of pentagons and heptagons (pentaheptite). ( n ), Calculated quantum capacitance (defined in the text) of perfect and polycrystalline/disordered graphene layers. Full size image Other than aqueous electrolyte, we also explored the use of an ionic-liquid electrolyte in our LIG-MSCs. Supplementary Fig. 14 shows CV and CC curves of LIG-MSCs in BMIM-BF 4 (1-butyl-3-methylimidazolium tetrafluoroborate), which suggest excellent capacitive behaviours. The corresponding specific-volumetric capacitances (C V ) versus discharge-volumetric current densities (I D ) is shown in Supplementary Fig. 15 . For practical applications requiring either higher operation potential or current or both, supercapacitors need to be connected in serial and/or parallel configurations. As shown in Supplementary Fig. 16 , the output potentials and currents can be well-controlled by serial and parallel connections to power the light-emitting diodes. Compared with commercial devices such as aluminium electrolytic capacitors, thin film Li-ion batteries, and activated-carbon supercapacitors, LIG-MSCs offer more energy or power density or both as seen from the Ragone plots ( Supplementary Fig. 17a ). When compared with recently demonstrated reduced GO-film (called MPG films [13] ) MSCs (MPG-MSCs) and laser-scribed graphene MSCs (LSG-MSCs) [18] , LIG-MSCs can deliver comparable E V , although power performance needs to be enhanced. Using specific areal energies (E A ) and power (P A ) densities, one can obtain reasonable values for comparing performance of in-plane MSCs intended for commercial applications. Supplementary Fig. 17b shows that LIG-MSCs exhibit ~100 × higher E A and ~4 × P A than MPG-MSCs. Furthermore, LIG-MSCs offer slightly better E A than LSG-MSCs with comparable power performance. In addition, cycling performance shows that there is negligible capacitance degrading after 9,000 cycles in aqueous electrolytes and 7,000 cycles in ionic-liquid electrolytes ( Supplementary Fig. 18 ). Moreover, CV curves at every 1,000 cycles show no involved pseudo-capacitive peaks ( Supplementary Fig. 19 ). The high capacitance of the LIG-MSC can be attributed to the 3D network of highly conductive graphene showing high surface area and abundant wrinkles, which provide easy access for the electrolyte to form a Helmholtz layer. Moreover, density function theory (DFT) calculations suggest that the ultra-polycrystalline nature of LIG-MSC can also improve the capacitance. The total capacitance ( C ) is determined by the quantum capacitance ( C q ), and the liquid electrolyte ( C l ) consisting of Helmholtz and diffusion regions [33] : C −1 = C q −1 + C l −1 . C l is mostly controlled by surface area. C q represents the intrinsic property of the electrode material and can be calculated from its electronic structure in equation (1) [34] : where S is the surface area, V is the applied voltage, D is the density of states, ε F is the Fermi level, and e is the electron charge. The ultra-polycrystalline nature suggested by Fig. 2c,d , as well as, Fig. 3d indicates the abundance of grain boundaries (GBs), which are composed of pentagon and heptagon pairs [35] . These defects are more ‘metallic’ than regular hexagons [36] , and therefore can be expected to enhance the charge storage performance. Calculations are performed by using DFT, with details elaborated in the Supplementary Methods . The GB effect is modelled by a planar polycrystalline graphene sheet ( Supplementary Fig. 20 ). Two types of GBs are considered as representatives ( Fig. 4j–k ). As an extreme case, we also consider a graphene sheet fully composed of pentagons and heptagons ( Fig. 4l ), so called ‘pentaheptite’ [37] . The calculated C q is shown in Fig. 4n . Clearly, a polycrystalline sheet has a much higher C q than perfect graphene, as a result of a higher density of states near the Fermi level owing to the presence of GBs. The type II GB enhances the storage more than in type I, as it has a higher defect density along the GBs. The highest C q is found in pentaheptite owing to its highest disorders and metallicity. Though here only the C q is calculated, it can be expected that the C tot increases as C q increases. These results suggest that GBs-rich LIG with maintained-electric conductivity would be able to deliver higher capacitance than perfect defect-free graphitic materials. Chemical doping of its rich ultra-polycrystalline domains of pentagon-heptagon rings might further enhance the capacitance. This is the first theoretical calculation that shows the effect of pentagon-heptagon grain boundaries on charge storage, a result that could inspire theoreticians to further explore the potential of these materials. In summary, we have developed a one-step and scalable approach to the preparation of porous graphene from commercial polymer sheets using CO 2 laser irradiation under ambient conditions. We have established that the physical and chemical properties of the resulting LIG structures render them uniquely suitable for energy storage devices delivering promising electrochemical performance. The use of commercially available polymer sheets would allow for roll-to-roll manufacturing, which bespeaks of ease in commercialization. Theoretical modelling suggests that the enhanced capacitance could partially come from defect-rich boundaries in LIG. This work might inspire both experimentalists and theoreticians to reexamine the potential of this technique in fields ranging from energy storage and conversion to electronics. Kapton PI (Cat. No. 2271K3, thickness: 0.005 inch) and other polymers sheets used in this work were all purchased from McMaster-Carr unless stated otherwise. They were used as received unless noted otherwise. Laser scribing on polymer sheets were conducted with a CO 2 laser cutter system (Universal X-660 laser cutter platform): 10.6 μm wavelength of laser with pulse duration of ~14 μs. The beam size is ~120 μm. Laser power was varied from 2.4 to 5.4 W with increments of 0.6 W. The laser system offers an option of controlling the scan rates from 0.7 to 23.1 inches s −1 . The laser system also provides an option of setting the pulses per inch (p.p.i.) with a range of 10–1,000 p.p.i. By experimentation it was discovered that the p.p.i. rate played little role in changing the threshold power. Other than as specifically stated, the same scan rate of 3.5 inch s −1 and 1,000 p.p.i. were used for all experiments. All of the laser experiments were performed under ambient conditions. Device fabrication LIG electrodes were directly written using the computer-controlled CO 2 laser. In the MSCs, the LIG serves as both the active electrodes and current collectors. For better electrical connection, silver paint was applied on the common areas of the positive and negative electrodes. The electrodes were extended with conductive copper tapes and then connected to electrochemical workstation. To protect the contact pads from the electrolyte, Kapton PI tape was employed to define the interdigitated area ( Fig. 4c ). Characterization SEM images were taken on a FEI Quanta 400 high resolution field emission instrument. The TEM and high-resolution TEM were performed using a 2,100 F field emission gun. Aberration-corrected scanning TEM images were taken using an 80 KeV JEOL ARM200F equipped with a spherical aberration corrector. The LIG films were peeled off and sonicated in chloroform before being transferred onto a C-flat TEM grid. XPS was performed using a PHI Quantera SXM Scanning X-ray Microprobe with a base pressure of 5 × 10 –9 Torr. All of the survey spectra were recorded in 0.5 eV step size with a pass energy of 140 eV. Elemental spectra were recorded in 0.1 eV step sizes with a pass energy of 26 eV. All the spectra were corrected using C1s peaks (284.5 eV) as references. XRD was conducted on a Rigaku D/Max ultima II with Cu Kα radiation (λ=1.54 Å). A Renishaw Raman microscope using 514-nm laser excitation at room temperature with a laser power of 5 mW was employed to obtain Raman spectra. A Nicolet infrared spectroscope was used to acquire the Fourier-transform infrared spectra. The surface area of LIG was measured with a Quantachrome autosorb-3b BET surface analyzer. Thermogravimetric analysis (Q50, TA Instruments) thermograms were carried out between 100–900 °C at 5 °C min −1 under argon; the water content was calculated from the weight loss between room temperature and 100 °C. The R s were measured using a Keithley four-point probe meter (model: 195 A, detection limit: 20 MΩ). The LIG samples for XRD, BET and thermogravimetric-analysis experiments were powder scratched from LIG films. Other characterizations were conducted directly on LIG films. The crystalline size (L c ) along the c axis and domain size in the a axis (L a ) and of LIG are calculated from the characteristics of the XRD (002) and (100) peaks using the equations (2) and (3), respectively [38] : where λ is the wavelength of the X-ray ( λ =1.54 Å) and B 1/2 (2 θ ) (in radian units) is the full width at half maximum of the peaks (200) and (100). Using Raman spectroscopic data, and calculating the crystalline size in the a axis (L a ) from the ratio of integrated intensity of the G peak ( I G ) and D peak ( I D ), the L a can be obtained by equation (4) [29] : where λ l is wavelength of the Raman laser ( λ l =514 nm). Measurements CV, galvanostatic CC measurements, and electrochemical impedance spectroscopy were performed using a CHI 608D workstation (USA). All of measurements were conducted in ambient conditions for aqueous electrolytes (1 M H 2 SO 4 ). The LIG-MSCs using 1-butyl-3-methylimidazolium tetrafluoroborate (BMIM-BF 4 , Sigma-Aldrich) were assembled and measured in an argon-filled glove box (VAC, model: NEXUS) with controlled O 2 and H 2 O levels lower than 1 p.p.m. To ensure full diffusion of ions onto surfaces of LIG electrodes, the microdevices were soaked in electrolyte for 2–3 h before measurements. electrochemical impedance spectroscopy was performed using the sinusoidal signal of 10 mV amplitude at a frequency ranging from 10 mHz–100 kHz. Calculation of parameters as indications for electrochemical performance of LIG-MSCs The specific areal capacitances ( C A , in mF·cm −2 ) based on the CV curves were calculated by equation (5): where S is the total surface area of active electrodes (in cm 2 ) with 0.6 cm 2 for the devices configuration used in this work; ν is the voltage sweep rate (in V·s −1 ); V f and V i are the potential limits of CV curves; and I ( V ) is the voltammetric current (in amperes). is the integrated area from CV curves. The total surface area of the device including the spacing between electrodes was ~0.86 cm 2 , which is used for calculating the power and energy density in the Ragone plot shown in Supplementary Fig. 17 . The specific areal ( C A , in mF cm −2 ) and volumetric capacitance ( C V , in F m −3 ) were calculated from the CC curves by equation (6) and (7) [10] : where I is the discharge current (in amperes) and d V /d t is the slope of galvanostatic discharge curves. S is the total area of the active positive and negative electrodes and d is the thickness of active materials. For the devices used in Supplementary Figs 15 and 17a , d was ~25 μm. The specific areal ( E A , in μWh cm −2 ) and volumetric energy densities ( E V , in Wh m −3 ) were calculated from equations (8) and (9): where Δ V=V max − V drop is the discharge potential range ( V max is the maximum voltage, 1 V for H 2 SO 4 , 3.5 V for BMIM-BF 4 ), V drop is the voltage drop indicated from the difference of the first two data points in the discharge curves. The specific areal ( P A , in mW cm 2 ) and volumetric ( P V , in W cm 3 ) power densities were obtained from equations (10) and (11): where Δ t is discharge time (in s). DFT calculations of perfect and polycrystalline graphene layers DFT calculations were performed with projector-augmented wave pseudopotentials and Perdew–Burke–Ernzerhof exchange-correlation functional, as implemented in VASP [39] , [40] . All structures were relaxed until the force on each atom was <0.01 eV Å −1 . Two types of polycrystalline sheets are considered, as shown in Supplementary Fig. 20 . Monkhorst-Pack k-points [41] sampling is used, with a vacuum space >15 Å in the non-periodic direction. To obtain the density of states, we use the tetrahedron method with Blöchl corrections [42] with a 45 × 7 × 1 k-points mesh. How to cite this article : Lin, J. et al. Laser-induced porous graphene films from commercial polymers. Nat. Commun. 5:5714 doi: 10.1038/ncomms6714 (2014).